Sensitive detection of proteasomal activation using the Deg-On mammalian synthetic gene circuit The ubiquitin proteasome system (UPS) has emerged as a drug target for diverse diseases characterized by altered proteostasis, but pharmacological agents that enhance UPS activity have been challenging to establish. Here we report the Deg-On system, a genetic inverter that translates proteasomal degradation of the transcriptional regulator TetR into a fluorescent signal, thereby linking UPS activity to an easily detectable output, which can be tuned using tetracycline. We demonstrate that this circuit responds to modulation of UPS activity in cell culture arising from the inhibitor MG-132 and activator PA28γ. Guided by predictive modelling, we enhanced the circuit’s signal sensitivity and dynamic range by introducing a feedback loop that enables self-amplification of TetR. By linking UPS activity to a simple and tunable fluorescence output, these genetic inverters will enable a variety of applications, including screening for UPS activating molecules and selecting for mammalian cells with different levels of proteasome activity. Protein homoeostasis in eukaryotic cells relies on the quality control function of the ubiquitin proteasome system (UPS), a complex macromolecular machinery that regulates protein turnover and catalyses degradation of misfolded or damaged proteins [1] . Protein degradation by the UPS involves covalent modification of substrates via polyubiquitin attachment [1] , [2] and degradation by the 26S proteasome [1] , [3] . UPS dysfunction has been linked to the pathogenesis of several diseases, ranging from cancer to cardiovascular and neurodegenerative disorders [4] , implicating the UPS as a molecular target for therapeutic intervention in a diverse range of human diseases [5] . Small molecules and peptides that inhibit the peptidase activities of the proteasome have been widely used to characterize the role of the UPS in maintaining protein homoeostasis [6] and transitioned to the clinic for treatment of cancer and inflammatory diseases [7] , [8] . On the other hand, pharmacological agents that increase UPS activity remain largely unexplored [9] , [10] , [11] , [12] , although this mode of regulation has great potential to ameliorate the phenotypes associated with the development of protein deposition diseases, such as Parkinson’s [13] , [14] and Huntington’s [15] , [16] . There is evidence that proteasome activity could be upregulated by overexpressing proteasomal subunits [15] , [17] , [18] , increasing E3 ligase expression [19] , [20] , [21] and modulating the rates of proteasomal conformational changes that are rate limiting for peptidase activity [22] , [23] . Unfortunately, the molecular mechanisms controlling total proteasomal activity in cells are not sufficiently understood to rationally design compounds that upregulate UPS activity. Current technologies for discovering and characterizing proteasome activators present a number of inherent limitations. In vitro assays based on the use of purified UPS components provide valuable information on the specificity of pharmacological agents [24] , [25] , but fail to recapitulate the complexity of the cellular quality control system in situ and preclude evaluating cell permeability, toxicity and off-target effects [25] . Reporter proteins engineered to function as model UPS substrates have been used to investigate proteasomal degradation in cells or in vivo [26] , [27] , [28] . While enabling detection of proteasome inhibition by yielding an increase in output signal, these reporters are not ideal to quantify proteasome activation because enhancement of UPS activity inevitably leads to a decrease in output signal, which is typically not appealing for high-throughput applications. To develop a mammalian cell-based platform to quantify proteasomal degradation that is amenable to high-throughput screening of UPS activators, we created a genetic circuit that interfaces with the natural proteasomal degradation machinery to convert modulation of UPS activity into an easily detectable output signal. We named this system ‘Degradation On’ (Deg-On) because it contains a reporter molecule (green fluorescence protein (GFP), signal output) that is negatively regulated by a tetracycline repressor (TetR) variant, which has been engineered to serve as a UPS substrate. The engineered repressor functions as a signal inverter and converts enhancement of proteasomal degradation—and the reduced, potentially undetectable cellular concentration of a proteasomal substrate—into an increase in GFP output. We show herein that the Deg-On system reports on modulation of UPS activity, and that the Deg-On output signal can be tuned by tetracycline dosage. We also use predictive modelling to improve the sensitivity and dynamic range of this circuit, thus generating a generalizable screening technology for the discovery or proteasome activators. In summary, we present here a genetic inverter that can be tuned for detecting the desired degree of UPS activation, thereby opening the way to the discovery of chemical and genetic regulators of UPS function as well as to quantitative in vivo analyses of proteasome activity. The Deg-On inverter for quantifying proteasomal activity To build a synthetic circuit for quantifying UPS activity, we constructed a genetic inverter [29] , [30] in which GFP transcription is under the control of a genetically encoded UPS substrate ( Fig. 1a ). We chose to use TetR, a negative transcriptional regulator derived from the Tn 10 bacterial transposon. TetR binds to the tetracycline operator (TO) in a tetracycline-dependent manner and has been widely applied to regulate gene transcription in eukaryotic cells [31] , [32] , [33] , [34] . In this study, TetR was rewired to function as a UPS substrate by fusion to a degradation tag (TetR-Deg). Specifically, two TetR-Deg variants were generated: TetR-ODC, based on the cODC degron tag [35] , [36] , which is the 37 amino acid carboxy-terminal sequence of ornithine decarboxylase, a substrate degraded via ubiquitin-independent proteasomal degradation [36] ; and TetR-CL1, based on the CL1 degron [27] , [37] , which is a 16 residue hydrophobic peptide that targets fusion proteins to ubiquitin-dependent proteasomal degradation [37] . 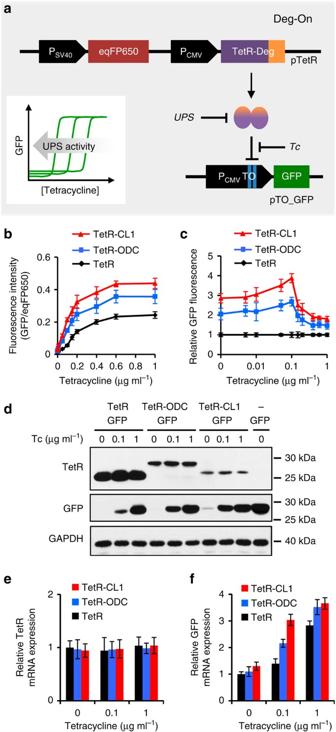Figure 1: The Deg-On system. (a) Schematic representation of the Deg-On system. The Deg-On system consists of two plasmids: pTetR encoding TetR-Deg and eqFP650 under the control ofPCMVandPSV40, respectively; and pTO_GFP encoding GFP under the control ofPCMV-TO. TetR-Deg is susceptible to proteasomal degradation and is displaced from TO by tetracycline (Tc). Both inputs (UPS activity andTc) enhance GFP expression. eqFP650 is independently and constitutively expressed from pTetR and serves as transfection control. By translating enhancement of UPS activity to increase in GFP fluorescence, TeR-Deg serves as UPS activity sensor and signal inverter, generating a positive correlation between UPS activity and GFP signal. Two distinct inputs (upregulation of UPS activity and tetracycline) generate the signal output (GFP fluorescence). Adjusting the tetracycline concentration allows tuning of circuit sensitivity to different degrees of UPS activation (inset). (b) Deg-On output signal as a function of tetracycline concentration. HeLa cells transfected with pTO_GFP and pTetR (encoding TetR, TetR-ODC or TetR-CL1) or with pTO_GFP and pTetR−were cultured with tetracycline (0–1 μg ml−1) for 30 h. GFP fluorescence intensities were normalized to those of eqFP650 (measured by flow cytometry) to correct for differences in transfection efficiency. The resulting values were divided by the fluorescence of control cells transfected with pTO_GFP and pTetR−and cultured without tetracycline. Data are reported as mean±s.d. (n≥3). (c) Relative Deg-On output signal as a function of tetracycline concentration. HeLa cells were transfected as described ina. Fluorescence intensities were normalized to those of cells transfected with pTO_GFP and pTetR encoding TetR lacking the degradation tag. (d) Western blot analyses of TetR and GFP in HeLa cells transfected with pTO_GFP and pTetR (encoding TetR, TetR-ODC, TetR-CL1) or with pTO_GFP and pTetR−and cultured with or without tetracycline for 30 h. GAPDH was used as a loading control. (e,f) Relative mRNA expression level of TetR (e) and GFP (f) in HeLa cells transfected as described ind. mRNA expression levels were evaluated by quantitative RT–PCR and normalized to those of the transfection control eqFP650. Data are reported as mean±s.d. (n=3). Figure 1: The Deg-On system. ( a ) Schematic representation of the Deg-On system. The Deg-On system consists of two plasmids: pTetR encoding TetR-Deg and eqFP650 under the control of P CMV and P SV40 , respectively; and pTO_GFP encoding GFP under the control of P CMV -TO. TetR-Deg is susceptible to proteasomal degradation and is displaced from TO by tetracycline ( T c). Both inputs (UPS activity and T c) enhance GFP expression. eqFP650 is independently and constitutively expressed from pTetR and serves as transfection control. By translating enhancement of UPS activity to increase in GFP fluorescence, TeR-Deg serves as UPS activity sensor and signal inverter, generating a positive correlation between UPS activity and GFP signal. Two distinct inputs (upregulation of UPS activity and tetracycline) generate the signal output (GFP fluorescence). Adjusting the tetracycline concentration allows tuning of circuit sensitivity to different degrees of UPS activation (inset). ( b ) Deg-On output signal as a function of tetracycline concentration. HeLa cells transfected with pTO_GFP and pTetR (encoding TetR, TetR-ODC or TetR-CL1) or with pTO_GFP and pTetR − were cultured with tetracycline (0–1 μg ml −1 ) for 30 h. GFP fluorescence intensities were normalized to those of eqFP650 (measured by flow cytometry) to correct for differences in transfection efficiency. The resulting values were divided by the fluorescence of control cells transfected with pTO_GFP and pTetR − and cultured without tetracycline. Data are reported as mean±s.d. ( n ≥3). ( c ) Relative Deg-On output signal as a function of tetracycline concentration. HeLa cells were transfected as described in a . Fluorescence intensities were normalized to those of cells transfected with pTO_GFP and pTetR encoding TetR lacking the degradation tag. ( d ) Western blot analyses of TetR and GFP in HeLa cells transfected with pTO_GFP and pTetR (encoding TetR, TetR-ODC, TetR-CL1) or with pTO_GFP and pTetR − and cultured with or without tetracycline for 30 h. GAPDH was used as a loading control. ( e , f ) Relative mRNA expression level of TetR ( e ) and GFP ( f ) in HeLa cells transfected as described in d . mRNA expression levels were evaluated by quantitative RT–PCR and normalized to those of the transfection control eqFP650. Data are reported as mean±s.d. ( n =3). Full size image To test whether each TetR-Deg retains tetracycline-dependent transcriptional repressor function, we evaluated GFP fluorescence as a function of tetracycline concentration (0–1 μg ml −1 medium concentration). This was achieved by transfecting HeLa cells with two plasmids encoding the Deg-On system: pTO_GFP, encoding GFP under the control of P CMV - TO ; and pTetR, encoding TetR or a TetR-Deg variant (TetR-ODC or TetR-CL1). A constitutively expressed far-red fluorescent protein (eqFP650 (ref. 38 ) was included in pTetR as a transfection control. GFP fluorescence increased with tetracycline concentration in cells expressing both TetR and TetR-Deg ( Fig. 1b ), indicating that the degron tags do not affect TetR binding to TO and tetracycline, as expected [39] . Moreover, cells expressing TetR-Deg displayed higher GFP fluorescence than cells expressing TetR at each tetracycline concentration tested, suggesting that the TetR variants accumulate to different cellular concentrations [40] and implicating the UPS in the degradation of TetR-Deg. The fluorescence of cells transfected with pTO_GFP and pTetR − (a pTetR derivative lacking the TetR gene) was observed not to depend on tetracycline concentration ( Supplementary Fig. 1a ), confirming that GFP expression depends on the cellular concentration of TetR as intended. Interestingly, the dynamic range of GFP signal on TetR-Deg degradation was found to vary with tetracycline concentration ( Fig. 1c ). We deduced that at low tetracycline concentrations, TO is partially occupied by TetR-Deg that is neither degraded nor displaced by tetracycline. Increasing tetracycline concentration in the culturing medium resulted in an increase in the relative GFP output until an optimum of tetracycline (0.1 μg ml −1 ), which corresponds to 3.9- and 2.7-fold increase in GFP fluorescence in cells expressing TetR-CL1 and TetR-ODC, respectively, compared with cells expressing TetR lacking a degradation tag. At higher tetracycline concentrations, the GFP signals from cells expressing TetR and TetR-Deg converge. This trend is interpreted as arising because tetracycline-induced displacement of TetR and TetR-Deg from TO prevails over degradation at high concentrations of tetracycline, impeding detection of proteasomal degradation using our genetic inverter. These data provide evidence that TetR-Deg degradation and tetracycline-induced displacement of TetR-Deg from TO occur independently and that these reactions simultaneously contribute to GFP expression levels. These data also show that tetracycline can be used to tune the sensitivity and dynamic range of the Deg-On system in response to UPS activity. Importantly, the fluorescence intensity of cells transfected with pTO_GFP and pTetR − was found to be considerably higher under steady-state conditions (30 h, Supplementary Fig. 1b ) than that of cells transfected with pTO_GFP and pTetR encoding TetR-ODC or TetR-CL1 (6.9- and 4.8-fold, respectively; Fig. 1b and Supplementary Fig. 1a ). This difference in output signal observed in the absence of TetR expression represents the theoretical maximal output signal arising from complete TetR degradation. To test whether the fluorescence signals detected by flow cytometry reflect TetR and GFP expression, we measured TetR and GFP protein levels. HeLa cells were transfected with pTO_GFP and each pTetR plasmid (encoding TetR, TetR-ODC or TetR-CL1) and treated with tetracycline (0, 0.1 and 1 μg ml −1 ), and TetR and GFP protein levels were evaluated by western blot. GFP accumulation increased proportionally with the concentration of tetracycline in cells expressing TetR or TetR-Deg ( Fig. 1d ), confirming that tetracycline regulates GFP expression. In contrast, tetracycline did not alter the accumulation of TetR or TetR-Deg. Moreover, the steady-state level of each TetR variant was inversely proportional to the GFP levels, with cells expressing TetR-CL1 presenting the lowest TetR and highest GFP concentration. These data confirm that TetR-Deg serves as a signal inverter. The largest increase in GFP accumulation in cells expressing TetR-Deg compared with cells expressing TetR was observed at 0.1 μg ml −1 tetracycline, in agreement with the results obtained by flow cytometry. As expected, cells transfected with pTO_GFP and pTetR − (lacking TetR) contained the highest level of GFP. To confirm that the changes in GFP fluorescence were due to post-translational regulation of TetR half-life and transcriptional regulation of GFP expression, we evaluated TetR and GFP messenger RNA levels using quantitative reverse transcription (RT)–PCR. We did not observe any significant change in TetR mRNA levels among cells expressing TetR or TetR-Deg treated with different concentrations of tetracycline ( Fig. 1e ), supporting our hypothesis that TetR, TetR-CL1 and TetR-ODC protein levels are regulated post translationally. However, we detected an increase in GFP mRNA levels in cells expressing TetR-Deg compared with cells expressing TetR ( Fig. 1f ), confirming that the Deg-On output signal arises from changes in transcriptional regulation of GFP. The Deg-On system is a sensor of UPS activation To evaluate whether the GFP output from the Deg-On circuit varies with UPS activity in cells, we examined the effect of the proteasome inhibitor MG-132 (ref. 6 ) on GFP expression within cells expressing TetR and each TetR-Deg. Specifically, HeLa cells were transfected with pTO_GFP and pTetR (encoding TetR, TetR-ODC or TetR-CL1) or with pTO_GFP and pTetR − (negative control). Transfected cells were cultured with tetracycline (0.1 μg ml −1 ) and MG-132 (3 μM). MG-132 treatment resulted in a 25 and 17% decrease in fluorescence in cells expressing TetR-ODC and TetR-CL1, respectively, compared with untreated cells ( Fig. 2a and Supplementary Fig. 2a ). However, MG-132 treatment did not affect the fluorescence of cells expressing TetR or lacking TetR ( Fig. 2a and Supplementary Fig. 2b ), suggesting that the Deg-On system provides an orthogonal circuit whose signal output can be used to quantify modulation of UPS activity. 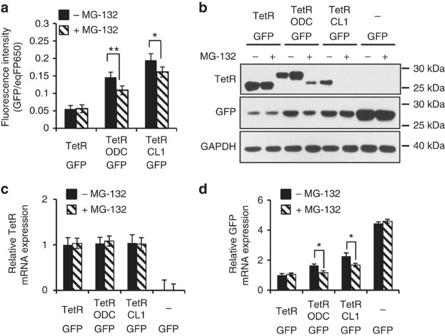Figure 2: Quantification of proteasomal degradation inhibition using the Deg-On system. HeLa cells transfected with pTO_GFP and pTetR (encoding TetR, TetR-ODC or TetR-CL1) or with pTO_GFP and pTetR−were treated with tetracycline 24 h post transfection (0.1 μg ml−1, 8 h), and subsequently exposed to tetracycline (0.1 μg ml−1) and MG-132 treatment (3 μM) for 16 h. (a) Deg-On output signal. GFP fluorescence intensity was normalized to that of eqFP650; the resulting fluorescence values were normalized to those of untreated cells transfected with pTO_GFP and pTetR−. Data are reported as mean±s.d. (n≥3, *P<0.05; **P<0.01, Student’st-test). (b) Western blot analyses of TetR and GFP. GAPDH was used as a loading control. (c,d) Relative mRNA expression level of TetR (c) and GFP (d). mRNA expression levels were evaluated by quantitative RT–PCR, corrected for the expression of the housekeeping geneGAPDHand normalized to those of the transfection control eqFP650. Data are presented as mean±s.d. (n=3, *P<0.05, Student’st-test). Figure 2: Quantification of proteasomal degradation inhibition using the Deg-On system. HeLa cells transfected with pTO_GFP and pTetR (encoding TetR, TetR-ODC or TetR-CL1) or with pTO_GFP and pTetR − were treated with tetracycline 24 h post transfection (0.1 μg ml −1 , 8 h), and subsequently exposed to tetracycline (0.1 μg ml −1 ) and MG-132 treatment (3 μM) for 16 h. ( a ) Deg-On output signal. GFP fluorescence intensity was normalized to that of eqFP650; the resulting fluorescence values were normalized to those of untreated cells transfected with pTO_GFP and pTetR − . Data are reported as mean±s.d. ( n ≥3, * P <0.05; ** P <0.01, Student’s t -test). ( b ) Western blot analyses of TetR and GFP. GAPDH was used as a loading control. ( c , d ) Relative mRNA expression level of TetR ( c ) and GFP ( d ). mRNA expression levels were evaluated by quantitative RT–PCR, corrected for the expression of the housekeeping gene GAPDH and normalized to those of the transfection control eqFP650. Data are presented as mean±s.d. ( n =3, * P <0.05, Student’s t -test). Full size image To directly evaluate the effect of MG-132 treatment on the Deg-On system output, we analysed TetR and GFP protein and mRNA levels. Western blot analyses revealed an increase in TetR protein levels in cells expressing TetR-ODC and TetR-CL1 treated with MG-132 compared with untreated cells ( Fig. 2b ), confirming that TetR-ODC and TetR-CL1 half-lives respond to modulation of proteasomal degradation. GFP accumulation was found to decrease in cells expressing TetR-ODC and TetR-CL1 treated with MG-132, compared with untreated cells. However, MG-132 treatment did not affect TetR and GFP protein levels in cells expressing TetR or lacking TetR. Quantitative RT–PCR analyses revealed that MG-132 does not cause significant changes in TetR mRNA levels in cells transfected with any of the TetR variants ( Fig. 2c ). GFP mRNA levels were found to be reduced on MG-132 treatment in cells expressing the TetR-Deg variants ( Fig. 2d ), but not in cells expressing TetR or lacking TetR. These results show that the Deg-On output signal depends on post-translational regulation of TetR half-life by the UPS and on transcriptional regulation of GFP by TetR. Modelling predicts improved sensitivity with feedback loop To predict variations in the Deg-On circuit’s architecture that would enhance the Deg-On output signal, we developed a mathematical model based on ordinary differential equations and quasi-steady-state assumptions that describes TetR and GFP concentrations (the parameter values are reported in the Supplementary Table 1 ). In this model, GFP and TetR expression were controlled by the rates of protein synthesis, degradation and cell dilution arising from cell division. Specifically, TetR synthesis was modelled as constitutive, while GFP production was dependent on the equilibrium between TetR and tetracycline-bound TetR as described in the Methods. This simplified model is based on the assumptions that TetR dissociation from DNA is a function of tetracycline concentration, with singly repressed promoter states ignored and that transcription is fast compared with translation as previously reported [41] . Our experimental data demonstrate that the GFP output of cells expressing TetR or TetR-Deg at high concentration of tetracycline reaches a plateau signal that is lower than the signal observed in cells expressing TO_GFP but lacking TetR ( Fig. 1b and Supplementary Fig. 1a ). To build a model that recapitulates our experimental results, which suggest residual repression of TO_GFP even at high concentrations of tetracycline as previously reported [33] , [42] , GFP expression was derived to include binding of tetracycline-bound TetR to TO, as described in the Methods. The predicted GFP expression at steady state increased as a function of tetracycline concentration and UPS activity, which was simulated by decreasing TetR half-life ( Fig. 3a ). The simulated GFP output as a function of tetracycline concentration and TetR half-life recapitulates the experimental results, with decreases in TetR half-life resulting in higher GFP signal intensity ( Fig. 3b ) and sensitivity ( Fig. 3c ). Our modelling also revealed that the concentration of tetracycline can be modulated to fine tune the sensitivity of the system ( Fig. 3c ). Low tetracycline concentration (0.05 μg ml −1 ) yielded a dramatic change in GFP expression with small changes in TetR half-life, whereas increasing tetracycline dosage (0.3 μg ml −1 ) lowers the output sensitivity to modulation of UPS activity. The agreement of our simulations with our experimental observations ( Figs 1 and 2 ) provides additional evidence that the Deg-On output signal reports on UPS activity. 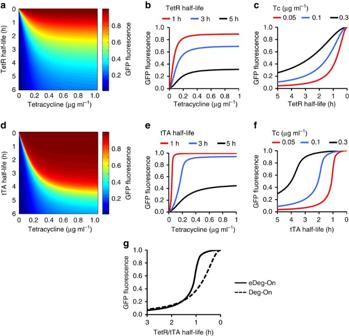Figure 3: Prediction of GFP output signal as a function of UPS activity and tetracycline dosage. GFP expression was predicted using the mathematical model described in the Methods. Relative GFP fluorescence values were calculated by normalizing GFP expression levels to those obtained in the absence of repressor. (a) Relative GFP output of the Deg-On system as a function of tetracycline concentration and TetR half-life. (b) Relative GFP output of the Deg-On system as a function of tetracycline concentration assuming TetR half-life of 1, 3 and 5 h. (c) Relative GFP output of the Deg-On system as a function of TetR half-life assuming cell exposure to 0.3, 0.1 and 0.05 μg ml−1tetracycline. (d) Relative GFP output of theeDeg-On system as a function of tetracycline concentration and tTA half-life. (e) Relative GFP output of theeDeg-On system as a function of tetracycline concentration assuming tTA half-life of 1, 3 and 5 h. (f) Relative GFP output of theeDeg-On system as a function of tTA half-life and assuming exposure to 0.3, 0.1 and 0.05 μg ml−1tetracycline. (g) Comparison of the predicted relative GFP output of theeDeg-On and Deg-On systems as a function of TetR half-life and assuming exposure to 0.05 μg ml−1tetracycline. Figure 3: Prediction of GFP output signal as a function of UPS activity and tetracycline dosage. GFP expression was predicted using the mathematical model described in the Methods. Relative GFP fluorescence values were calculated by normalizing GFP expression levels to those obtained in the absence of repressor. ( a ) Relative GFP output of the Deg-On system as a function of tetracycline concentration and TetR half-life. ( b ) Relative GFP output of the Deg-On system as a function of tetracycline concentration assuming TetR half-life of 1, 3 and 5 h. ( c ) Relative GFP output of the Deg-On system as a function of TetR half-life assuming cell exposure to 0.3, 0.1 and 0.05 μg ml −1 tetracycline. ( d ) Relative GFP output of the e Deg-On system as a function of tetracycline concentration and tTA half-life. ( e ) Relative GFP output of the e Deg-On system as a function of tetracycline concentration assuming tTA half-life of 1, 3 and 5 h. ( f ) Relative GFP output of the e Deg-On system as a function of tTA half-life and assuming exposure to 0.3, 0.1 and 0.05 μg ml −1 tetracycline. ( g ) Comparison of the predicted relative GFP output of the e Deg-On and Deg-On systems as a function of TetR half-life and assuming exposure to 0.05 μg ml −1 tetracycline. Full size image We next used our model to predict strategies that enhance the dynamic range and sensitivity of the Deg-On circuit. As previous studies demonstrated a linearizing effect of negative feedback-based gene circuits [41] , [43] , we hypothesized that engineering TetR-Deg to function as a self-activator would result in a positive feedback loop that, in turn, would enhance the Deg-On output signal sensitivity to modulation of UPS activity [44] . A positive feedback loop can be introduced in the Deg-On system by controlling GFP output using the tetracycline-controlled transactivator (tTA), which consists of TetR fused to the transcriptional activator domain VP16 (ref. 34 ). Similar to TetR, tTA functions as a repressor when bound to a TO that is placed downstream of the promoter TATA box [33] . In contrast to TetR, however, tTA can additionally function as an activator when bound to a TO that is placed upstream of a minimal CMV promoter, for example, P TRE , which consists of seven TO cassettes upstream of a minimal CMV promoter [34] . We envisioned introducing a feedback loop into the Deg-On system by including two tTA-encoding genes, one under control of an inducible promoter ( P TRE ) that results in self-activated expression and the other under control of a constitutive promoter ( P CMV ) that initiates the self-activation loop (as described in the Methods). Mathematical modelling of GFP expression from this ‘enhanced Deg-On’ ( e Deg-On) system revealed that, on addition of the self-amplification loop, the output signal still responds to tetracycline dosage and UPS activity ( Fig. 3d ). GFP expression in the e Deg-On system is predicted to depend on tTA half-life in the presence of different tetracycline concentrations ( Fig. 3e,f ), like in the Deg-On system, but the greater e Deg-On output signal sensitivity to changes in the repressor half-life suggests that this alternative architecture enables more precise detection of UPS activation. To directly compare the UPS dependence of the Deg-On and e Deg-On system outputs, we simulated GFP expression as a function of TetR and tTA half-life, respectively, under constant tetracycline dosing conditions (0.05 μg ml −1 ). We observed a considerably sharper increase in the e Deg-On output signal compared with the Deg-On output signal at TetR half-lives between 1 and 2 h ( Fig. 3g ), implicating the e Deg-On system as having a greater sensitivity to modulation of UPS activity. Interestingly, the e Deg-On system is predicted to lose sensitivity at high UPS activity (TetR half-life below 1 h). Under these conditions, lower tetracycline concentrations can be used to tune the system and allow for detection of UPS activation ( Fig. 3e,f ). e Deg-On displays enhanced sensitivity UPS activation To experimentally test whether the e Deg-On system exhibits improved sensitivity as predicted, we constructed two tTA variants that function as UPS substrates (tTA-Deg), consisting of tTA fused to the CL1 (tTA-CL1) or the ODC (tTA-ODC) tag. A three-plasmid system was used to implement the e Deg-On system, including pTRE_tTA encoding tTA or tTA-Deg under the control of P TRE ; ptTA encoding tTA or tTA-Deg under the control of P CMV ; and pTO_GFP encoding GFP under the control of P CMV - TO ( Fig. 4a ). We hypothesized that constitutive expression of tTA-Deg from ptTA would result in induction of the self-activation loop from pTRE_tTA as well as repression of GFP expression from pTO. The optimal pTRE_tTA to ptTA ratio for transfection was experimentally determined ( Supplementary Fig. 3 ). 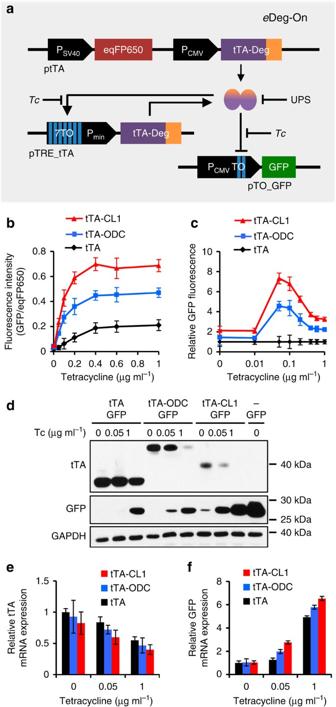Figure 4: TheeDeg-On system. (a) Schematic representation of theeDeg-On system. TheeDeg-On system consists of three plasmids: ptTA encoding tTA-Deg and eqFP650 under the control of thePCMVandPSV40, respectively; pTO_GFP encoding GFP under the control ofPCMV-TO; and pTRE_tTA encoding tTA-Deg under the control ofPTRE(7TO_Pmin), and eqFP650 under the control ofPSV40(not shown). tTA-Deg is a sensor of UPS activity and a repressor of GFP expression. tTA-Deg activates its own expression by binding toPTREand is also constitutively expressed from ptTA. (b)eDeg-On output signal as a function of tetracycline concentration. HeLa cells transfected with pTO_GFP, ptTA and pTRE_tTA (encoding tTA, tTA-ODC or tTA-CL1) or with pTO_GFP and pTetR−were cultured with tetracycline (0–1 μg ml−1) for 30 h. Cell fluorescence was measured and analysed as described inFig. 1b. Data are reported as mean±s.d. (n≥3). (c) RelativeeDeg-On output signal as a function of tetracycline concentration. HeLa cells were transfected as described ina. Fluorescence intensities were normalized to those of cells transfected with pTO_GFP, ptTA and pTRE_tTA encoding tTA lacking the degradation tag to evaluate the relative increase in output signal associated with expression of a tTA-Deg variant. (d) Western blot analyses of tTA and GFP in HeLa cells transfected with theeDeg-On system as described ina. GAPDH was used as a loading control. (e,f) Relative mRNA expression level of tTA (e) and GFP (f) in HeLa cells transfected with theeDeg-On system as described ina. mRNA expression levels were evaluated by quantitative RT–PCR, corrected for the expression of the housekeeping geneGAPDHand normalized to those of the transfection control eqFP650. Data are reported as mean±s.d. (n=3). Figure 4: The e Deg-On system. ( a ) Schematic representation of the e Deg-On system. The e Deg-On system consists of three plasmids: ptTA encoding tTA-Deg and eqFP650 under the control of the P CMV and P SV40 , respectively; pTO_GFP encoding GFP under the control of P CMV -TO; and pTRE_tTA encoding tTA-Deg under the control of P TRE (7TO_ P min ), and eqFP650 under the control of P SV40 (not shown). tTA-Deg is a sensor of UPS activity and a repressor of GFP expression. tTA-Deg activates its own expression by binding to P TRE and is also constitutively expressed from ptTA. ( b ) e Deg-On output signal as a function of tetracycline concentration. HeLa cells transfected with pTO_GFP, ptTA and pTRE_tTA (encoding tTA, tTA-ODC or tTA-CL1) or with pTO_GFP and pTetR − were cultured with tetracycline (0–1 μg ml −1 ) for 30 h. Cell fluorescence was measured and analysed as described in Fig. 1b . Data are reported as mean±s.d. ( n ≥3). ( c ) Relative e Deg-On output signal as a function of tetracycline concentration. HeLa cells were transfected as described in a . Fluorescence intensities were normalized to those of cells transfected with pTO_GFP, ptTA and pTRE_tTA encoding tTA lacking the degradation tag to evaluate the relative increase in output signal associated with expression of a tTA-Deg variant. ( d ) Western blot analyses of tTA and GFP in HeLa cells transfected with the e Deg-On system as described in a . GAPDH was used as a loading control. ( e , f ) Relative mRNA expression level of tTA ( e ) and GFP ( f ) in HeLa cells transfected with the e Deg-On system as described in a . mRNA expression levels were evaluated by quantitative RT–PCR, corrected for the expression of the housekeeping gene GAPDH and normalized to those of the transfection control eqFP650. Data are reported as mean±s.d. ( n =3). Full size image To test whether tTA-Deg in the e Deg-On system functions as predicted, we measured the fluorescence of HeLa cells transfected with pTO_GFP, ptTA and pTRE_tTA as a function of tetracycline concentration. GFP fluorescence increased as a function of tetracycline concentration, confirming that tTA-Deg retains tetracycline-dependent repressor activity ( Fig. 4b ). Cells expressing tTA-CL1 and tTA-ODC displayed 2.1- and 1.4-fold higher fluorescence, respectively, than cells expressing tTA at tetracycline concentrations between 0 and 0.01 μg ml −1 . The fluorescence of cells expressing these tTA-Deg variants further increased to 7.3- and 4.5-fold higher fluorescence at tetracycline concentrations between 0.05 and 0.1 μg ml −1 ( Fig. 4c ). We concluded that the addition of 0.05 μg ml −1 of tetracycline to the culturing medium is optimal to detect even limited increase in UPS activity and thus results in maximal output dynamic range and sensitivity in response to tTA degradation. The kinetics of tetracycline induction in the e Deg-On system ( Supplementary Fig. 4a ) was similar to that observed in the Deg-On system ( Supplementary Fig. 1b ). These results suggest that self-amplification of the UPS sensor enhances the sensitivity of the gene circuit and amplifies the dynamic range of the output signal ( Supplementary Fig. 4b–d ), validating the prediction of the mathematical model. To verify that the GFP signal in the e Deg-On system is linked to tTA self-activation, we measured tTA and GFP protein and mRNA levels in HeLa cells expressing the e Deg-On system. We found that tTA and tTA-Deg protein concentrations ( Fig. 4d ) and mRNA levels ( Fig. 4e ) decreased with increasing tetracycline concentration, confirming that tTA-Deg self-activation is negatively regulated by tetracycline. We also observed an increase in GFP protein concentration ( Fig. 4d ) and mRNA levels ( Fig. 4f ) on increase in tetracycline dosage. Importantly, GFP mRNA levels in cells exposed to high tetracycline concentrations (1 μg ml −1 ) were found to be 5- to 6.5-fold higher than those of untreated cells ( Fig. 4f )—a relative increase that is more than 2-fold higher than what we observed with the Deg-On system ( Fig. 1f ), demonstrating an enhanced dynamic range of the e Deg-On system. To confirm that the differences in GFP expression observed between the Deg-On and the e Deg-On system result from the introduction of the self-activation loop and are not caused by differences in TO-binding affinities between TetR and tTA, we compared the fluorescence of cells transfected with the e Deg-On system (pTRE_tTA, ptTA and pTO_GFP) with that of cells expressing the TetR-based Deg-On system (pTetR and pTO_GFP) or the tTA-based Deg-On system (ptTA and pTO_GFP). We did not observe significant differences between the output signals of TetR-based and tTA-based Deg-On systems ( Supplementary Fig. 5a,b ), which were both significantly lower than the output of the e Deg-On system ( Supplementary Figs 4b–d and 5 ). These results demonstrate that (i) the VP16 transcriptional activation domain does not influence tTA function as a transcriptional repressor and (ii) the transcriptional feedback loop mediates the signal amplification observed in the e Deg-On system. To verify that the e Deg-On system responds to modulation of UPS activity, we evaluated the output signal response to inhibition of proteasomal degradation. HeLa cells were transfected with the e Deg-On system and cultured with tetracycline (0.05 μg ml −1 ) and MG-132 (3 μM). On treatment with MG-132, cells expressing tTA-ODC and tTA-CL1 presented a 40 and 25% decrease in GFP fluorescence intensity, respectively ( Fig. 5a and Supplementary Fig. 6a ). The dynamic range of the e Deg-On output signal in response to MG-132 treatment was considerably higher than that of the Deg-On system under the same conditions (25 and 17%, respectively; Fig. 2a ), confirming that self-amplification of the UPS sensor enhances the circuit sensitivity to modulation of proteasomal degradation. 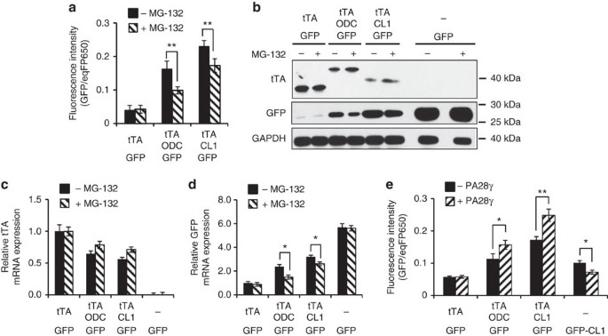Figure 5: Quantification of UPS modulation using theeDeg-On system. (a) HeLa cells transfected with pTO_GFP, ptTA, pTRE_tTA (encoding tTA, tTA-ODC or tTA-CL1) or with pTO_GFP and pTetR−were treated with tetracycline 24 h post transfection (0.05 μg ml−1, 8 h), and subsequently exposed to tetracycline (0.05 μg ml−1) and MG-132 treatment (3 μM) for 16 h. (a)eDeg-On output signal on inhibition of proteasomal degradation. GFP fluorescence intensity was normalized to that of eqFP650; the resulting fluorescence values were normalized to those of untreated cells transfected with pTO_GFP and pTetR−. Data are reported as mean±s.d. (n≥3, **P<0.01, Student’st-test). (b) Western blot analyses of tTA and GFP. GAPDH was used as a loading control. (c,d) Relative mRNA expression level of tTA (c) and GFP (d). mRNA expression levels were evaluated by quantitative RT–PCR, corrected for the expression of the housekeeping geneGAPDHand normalized to those of the transfection control eqFP650. Data are presented as mean±s.d. (n=3, *P<0.05, Student’st-test). (e)eDeg-On output signal on activation of proteasomal degradation. HeLa cells transfected with (i) pTO_GFP, ptTA, pTRE_tTA (encoding tTA, tTA-ODC or tTA-CL1), with pTO_GFP and pTetR−or with pTO_GFP-CL1 and with (ii) pPA28, a pcDNA3.1 derivative encoding PA28γ, or pcDNA3.1, were treated with tetracycline 24 h post transfection (0.05 μg ml−1, 24 h). GFP fluorescence intensity was normalized to that of eqFP650; the resulting fluorescence values were normalized to those of cells transfected with pTO_GFP, pTetR−and pcDNA3.1. Data are presented as mean±s.d. (n=3, *P<0.05; **P<0.01, Student’st-test). Figure 5: Quantification of UPS modulation using the e Deg-On system. ( a ) HeLa cells transfected with pTO_GFP, ptTA, pTRE_tTA (encoding tTA, tTA-ODC or tTA-CL1) or with pTO_GFP and pTetR − were treated with tetracycline 24 h post transfection (0.05 μg ml −1 , 8 h), and subsequently exposed to tetracycline (0.05 μg ml −1 ) and MG-132 treatment (3 μM) for 16 h. ( a ) e Deg-On output signal on inhibition of proteasomal degradation. GFP fluorescence intensity was normalized to that of eqFP650; the resulting fluorescence values were normalized to those of untreated cells transfected with pTO_GFP and pTetR − . Data are reported as mean±s.d. ( n ≥3, ** P <0.01, Student’s t -test). ( b ) Western blot analyses of tTA and GFP. GAPDH was used as a loading control. ( c , d ) Relative mRNA expression level of tTA ( c ) and GFP ( d ). mRNA expression levels were evaluated by quantitative RT–PCR, corrected for the expression of the housekeeping gene GAPDH and normalized to those of the transfection control eqFP650. Data are presented as mean±s.d. ( n =3, * P <0.05, Student’s t -test). ( e ) e Deg-On output signal on activation of proteasomal degradation. HeLa cells transfected with (i) pTO_GFP, ptTA, pTRE_tTA (encoding tTA, tTA-ODC or tTA-CL1), with pTO_GFP and pTetR − or with pTO_GFP-CL1 and with (ii) pPA28, a pcDNA3.1 derivative encoding PA28γ, or pcDNA3.1, were treated with tetracycline 24 h post transfection (0.05 μg ml −1 , 24 h). GFP fluorescence intensity was normalized to that of eqFP650; the resulting fluorescence values were normalized to those of cells transfected with pTO_GFP, pTetR − and pcDNA3.1. Data are presented as mean±s.d. ( n =3, * P <0.05; ** P <0.01, Student’s t -test). Full size image To directly evaluate the effect of MG-132 treatment on the e Deg-On system output, we analysed tTA and GFP protein and mRNA levels. Western blot analyses revealed an increase in tTA and decrease in GFP protein concentrations in cells expressing tTA-Deg treated with MG-132, compared with untreated cells ( Fig. 5b ). As expected, MG-132 treatment altered neither tTA nor GFP protein levels in cells expressing unmodified tTA or lacking tTA ( Fig. 5b ). Moreover, tTA mRNA levels were found to increase on MG-132 treatment in cells expressing tTA-Deg, but not in cells expressing tTA ( Fig. 5c ), confirming that tTA-Deg transcription is self-activated and, as a result, is upregulated on increase in tTA-Deg half-life by MG-132 inhibition of the UPS. Accordingly, GFP mRNA levels were found to decrease on MG-132 treatment in cells expressing tTA-Deg, but not in cells expressing tTA or lacking tTA ( Fig. 5d ). To evaluate whether the extent of tTA-Deg aggregation [27] , particularly on proteasomal inhibition, contributes to the e Deg-On system output signal, we calculated the aggregation propensity factor (APF; see Methods) of HeLa cells transfected with the e Deg-On system, untreated or treated with MG-132, compared with control cells lacking both the tTA and GFP genes ( Supplementary Fig. 6b ). In the absence of MG-132, we did not observe significant differences among the APF of cells expressing tTA, tTA-Deg or lacking tTA, suggesting that under the expression conditions used in this study, the ODC and CL1 tags do not alter the aggregation propensity of tTA. On treatment with MG-132, we observed a 60% increase in APF with each condition ( P <0.05, Student’s t -test), reflecting the impact of proteasomal inhibition on the extent of total cellular protein aggregation. However, cells expressing the e Deg-On system presented an MG-132 induced increase in APF comparable to that of cells expressing only GFP, providing evidence that overexpression of tTA and tTA-Deg do not alter the extent of total protein aggregation. In summary, these results demonstrate that the e Deg-On output signal depends on the extent of tTA-Deg proteasomal degradation and not on the extent of tTA-Deg aggregation. To evaluate whether the e Deg-On system can serve as a quantitative reporter for enhancement of proteasomal degradation, we evaluated the e Deg-On output signal on genetic activation of UPS activity achieved by overexpressing the proteasome activator subunit PA28γ [15] . To this end, HeLa cells were transfected with the e Deg-On system and with a vector encoding PA28γ, and cultured with 0.05 μg ml −1 tetracycline. Overexpression of PA28γ resulted in a 38 and 44% increase in fluorescence intensity in cells expressing tTA-ODC and tTA-CL1, respectively, but did not affect the output signal of cells expressing tTA or lacking of tTA ( Fig. 5e and Supplementary Fig. 7 ). To compare the e Deg-On with a reporter system that directly links output signal to UPS activity [27] , [37] , we also tested HeLa cells expressing a GFP variant fused to a degron tag. Specifically, GFP was fused to the CL1 tag, which was found to result in highest dynamic range in the context of both Deg-On and e Deg-On systems. HeLa cells were transfected for the expression of GFP-CL1 system (ptTA − and pTO_GFP-CL1) and PA28γ (pPA28 or pcDNA3.1) and cultured under the same conditions used to test the e Deg-On system ( Fig. 5e ). The GFP output signal was found to decrease on overexpression of PA28γ as expected, confirming that the increase in PA28γ expression results in enhanced degradation of the CL1-tagged reporter. UPS activation resulted in 28% decrease in fluorescence intensity in cells expressing PA28γ, which is smaller than the increase elicited with the eDeg-On system. While this decrease was statistically significant ( P <0.05, Student’s t -test), the significance level obtained with a similar eDeg-On experiment ( P <0.01, Student’s t -test) was smaller. These findings suggest that the e Deg-On is likely to provide a more ideal circuit for detection of UPS activation because it provides a more sensitive system to translate the enhancement of proteasomal degradation into increase in signal output. In addition, these findings illustrate how the GFP-Deg system could provide a powerful couterscreen to validate hits selected in the context of the e Deg-On system that alter TetR-Deg degradation and eliminate potential false positives that arise from molecules that directly alter the expression level of the system components, for example, GFP. Such false positives would increase the signal obtained from both eDeg-On and GFP-Deg systems rather than eliciting opposite effects on the GFP signal as observed with PA28γ overexpression. To create a more robust platform for the detection of UPS modulation, we generated a stable cell line expressing the e Deg-On system. HEK293 were first transfected with pTO_GFP and a stable monoclonal population selected for transfection with ptTA and pTRE_tTA encoding the CL1-tagged tTA variant. To test whether the e Deg-On stable cell line recapitulates the features of the transiently transfected e Deg-On system, we monitored the effect of tetracycline dosage on the GFP output signal as well as the GFP and tTA protein levels. GFP fluorescence increased as a function of tetracycline concentration, displaying a range of signal increases (1.5- to 12-fold) between tetracycline concentrations of 0.01 and 1 μg ml −1 , respectively ( Fig. 6a ). We also found that tTA protein levels in the stable cell line decreased with increasing tetracycline concentration, confirming that tTA-CL1 self-activation is negatively regulated by tetracycline. As expected, GFP protein concentration increased with tetracycline dosage in the e Deg-On stable cell line, but did not depend on tetracycline in the parental stable cell line transfected only for the expression of GFP ( Fig. 6b ). The response of the e Deg-On stable cell line to modulation of UPS function was investigated using the proteasome inhibitor MG-132. MG-132 treatment decreased the output signal of the e Deg-On stable cell line by 38% ( Fig. 6c ) but did not affect the output signal of the parental clone stably transfected for the expression of GFP alone ( Supplementary Fig. 8a ). To confirm that the e Deg-On stable cell line is generally sensitive to chemical inhibition of proteasomal degradation, we also tested the output signal response to lactacystin, another well-established proteasome inhibitor [6] . Lactacystin treatment resulted in a 22% decrease in GFP fluorescence ( Fig. 6c and Supplementary Fig. 8a ), confirming that the e Deg-On stable cell line is a reliable sensor of proteasomal inhibition. Finally, to evaluate the use of the e Deg-On stable cell line as a sensor of proteasomal enhancement, we induced overexpression of the proteasome activator subunit PA28γ. Overexpression of PA28γ yielded a 31% increase in fluorescence output in the e Deg-On stable cell line but did not affect the output signal of the parental line expressing only GFP ( Fig. 6d and Supplementary Fig. 8b ). These results demonstrate that the e Deg-On system is a reliable sensor of UPS activation and a novel tool to quantify enhancement of proteasomal degradation. 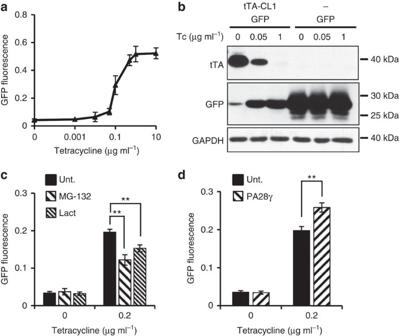Figure 6: Quantification of UPS modulation using a stableeDeg-On cell line. (a) A stable monoclonal populations of cells transfected for the expression of theeDeg-On system (PCMV-TO_GFP,PCMV-tTA-CL1 andPTRE_tTA-CL1) and the stable parental line transfected only for the expression of GFP (PCMV-TO_GFP) were treated with tetracycline for 36 h. The GFP fluorescence of cells expressing theeDeg-On system was normalized to that of the parental clone in which GFP is expressed constitutively. Data are presented as mean±s.d. (n=3). (b) Western blot analyses of tTA and GFP. GAPDH was used as a loading control. (c)eDeg-On output signal on inhibition of proteasomal degradation. The stable cell lines used inawere cultured with tetracycline (0 or 0.2 μg ml−1) and MG-132 (1 μM) or lactacystin (2 μM) for 24 h. The GFP fluorescence of cells expressing theeDeg-On system was normalized to that of the parental clone in which GFP was expressed constitutively. Data are presented as mean±s.d. (n=3, **P<0.01, Student’st-test). (d)eDeg-On output signal on activation of proteasomal degradation. The stable cell lines used inawere transfected with pPA28 or pcDNA3.1 and were treated with tetracycline 24 h post transfection (0 or 0.2 μg ml−1, 24 h). The GFP fluorescence of cells expressing theeDeg-On system was normalized to that of the parental clone in which GFP was expressed constitutively. Data are presented as mean±s.d. (n=3, **P<0.01, Student’st-test). Figure 6: Quantification of UPS modulation using a stable e Deg-On cell line. ( a ) A stable monoclonal populations of cells transfected for the expression of the e Deg-On system ( P CMV -TO_GFP , P CMV -tTA-CL1 and P TRE _tTA-CL1 ) and the stable parental line transfected only for the expression of GFP ( P CMV -TO_GFP ) were treated with tetracycline for 36 h. The GFP fluorescence of cells expressing the e Deg-On system was normalized to that of the parental clone in which GFP is expressed constitutively. Data are presented as mean±s.d. ( n =3). ( b ) Western blot analyses of tTA and GFP. GAPDH was used as a loading control. ( c ) e Deg-On output signal on inhibition of proteasomal degradation. The stable cell lines used in a were cultured with tetracycline (0 or 0.2 μg ml −1 ) and MG-132 (1 μM) or lactacystin (2 μM) for 24 h. The GFP fluorescence of cells expressing the e Deg-On system was normalized to that of the parental clone in which GFP was expressed constitutively. Data are presented as mean±s.d. ( n =3, ** P <0.01, Student’s t -test). ( d ) e Deg-On output signal on activation of proteasomal degradation. The stable cell lines used in a were transfected with pPA28 or pcDNA3.1 and were treated with tetracycline 24 h post transfection (0 or 0.2 μg ml −1 , 24 h). The GFP fluorescence of cells expressing the e Deg-On system was normalized to that of the parental clone in which GFP was expressed constitutively. Data are presented as mean±s.d. ( n =3, ** P <0.01, Student’s t -test). Full size image Enhancing the UPS capacity to dispose of misfolded, aggregation-prone proteins holds potential for the treatment of a range of protein misfolding diseases in which the formation of non-native proteinaceous inclusion bodies is associated with neurodegeneration [13] , [14] , [15] , [16] . Cellular proteasome activators, such as the proteasome subunits PA28, PA200 and PA700 are involved in fundamental cellular processes including antigen presentation and tumorigenesis [23] . Interestingly, overexpression of PA28γ was shown to recover proteasome function in an in vitro model of Huntington disease and improve cell viability [15] . Pharmacological agents that enhance UPS activity, however, are extremely rare: oleuropein was shown to enhance all three proteasome peptidase activities in fibroblasts [11] , while betulinic acid activates preferentially the chymotrypsin-like proteasome activity [9] and displays potentially anti-cancer properties [10] , [45] . Inhibition of the deubiquitinating enzyme USP14 was shown to enhance degradation of oxidized proteins, thereby protecting from oxidative stress [12] . The discovery and characterization of compounds that enhance proteasomal degradation has been generally hindered by the current lack of cell-based technologies to quantify enhancement of UPS activity. To address this need, we generated a cell-based technology that couples a synthetic gene circuit that senses inputs caused by modulation of UPS activity, to the cell’s natural regulatory circuitry, which produces an easily detectable fluorescent output. To build this genetic inverter, TetR was engineered to function as a substrate for the UPS and used to control the transcription of a fluorescent reporter. This genetic sensor was designed to sense inputs that culminate in UPS modulation, including intracellular inputs, such as altered expression of the proteasome activator subunit PA28γ, as well as extracellular inputs, such as exposure to small molecule proteasome inhibitors. While genetic circuits have been previously employed as screens for drug discovery [46] , this is the first evidence of an orthogonal circuit that interfaces specifically with the mammalian UPS machinery. TetR was rewired to function as a UPS substrate by fusion to two representative protein domains that are actively targeted to proteasomal degradation: the C terminus of ODC and the CL1 degron. Owing to the specific nature of these degradation sequences, our synthetic circuit can be tuned to interface with different proteasomal degradation pathways. Circuits containing TetR-ODC can be used to interface with a ubiquitin-independent pathway that mediates proteasomal degradation in collaboration with antizyme [36] , whereas TetR-CL1 can be used to report on the ubiquitin-dependent pathway that mediates proteasomal degradation via the Ubc6p-Ubc7p ubiquitin-conjugating enzyme pair [37] . Fusion of degradation tags to reporter protiens can afford precise control over the reporter protein’s turnover rate [47] . We expect that the ability to alter the sequence of degradation tag will make it possible to customize this genetic sensor for the discovery and characterization of different classes of proteasome activators. Moreover, we anticipate that altering the sequence specificity of the degradation tag will allow modulating the half-life of the engineered TetR, as previoulsy shown for other CL1 fusion proteins [37] . Thus, the interface between the engineered gene circuit and the cell’s regulatory circuitry could be further adapted for the discovery of proteasome modulators that display different activation kinetics by using TetR variants with desired degradation properties. To enhance the sensitivity and dynamic range of this orthogonal circuit and engineer a more robust and decisive cellular behaviour in response to modulation of UPS activity, we introduced a positive feedback loop that enables self-activation of the engineered TetR. Artificial positive feedback loops have been employed as genetic amplifiers for enhancing promoter activity [44] , [48] , [49] . In this study, addition of a positive feedback loop to amplify expression of the engineered TetR resulted in enhanced sensitivity of the gene circuit—defined as the slope of the relationship between output and input—to modulation of UPS activity. The predictive model described herein could be used to explore alternative or additional variations in the circuit’s architecture for customizing or further improving the dynamic range of the system. Whether stochasticity of gene expression leading to phenotypically distinct subpopulations affects the sensitivity of the e Deg-On system to changes in UPS activity, however, remains to be established [50] and optimization of the parts may be ultimately needed to ensure functionality in different biological settings [43] . The UPS plays an essential role in regulating a wide variety of fundamental cellular processes, including cell cycle, DNA repair, immune response and apoptosis [51] . Proteasome inhibitors have been widely used to characterize the UPS function and enabled dissection of important cellular pathways involved in the degradation of misfolded proteins, cell cycle, inflammatory and immune response, disease development, metabolism, circadian rhythms, photomorphogenesis and muscle atrophy [6] . The activity of proteasome inhibitors as anti-cancer, anti-inflammatory, angiostatic and immunomodulating agents was reported [6] , and their clinical potential as cancer chemotherapeutics has been amply documented [7] , [52] , [53] . Particularly, bortezomib (Velcade) was the first proteasome inhibitor to be tested in humans and is approved for the treatment of multiple myeloma and mantle cell lymphoma [54] . While evidence of the molecular mechanisms that could be potentially targeted to enhance UPS activity is emerging [12] , [13] , [17] , [18] , [19] , [20] , [21] , [22] , [23] , it remains challenging to rationally design compounds that activate proteasomal degradation. The genetic circuits reported herein should be generally useful for in vitro and in vivo investigations aimed at deciphering the cellular regulatory networks that underlie modulation of UPS function in different cell types. The input–output behaviour of the e Deg-On system was also confirmed in the context of stable cell lines generated by genetically integrating the relevant parts of the circuits ( P TRE _tTA-CL1 , P CMV _tTA-CL1 and P CMV - TO_GFP ) into the chromosome. By providing a cell-based platform to quantify modulation of UPS activity, this e Deg-On cell line may also find applications in the screening for compounds that enhance UPS activity, which, in turn, will open the way to the development of therapeutic strategies to reduce the accumulation of aberrant proteins under conditions of proteotoxic stress. Primers and plasmids The cloning primers are listed in Supplementary Table 2 . pTO_GFP was constructed by cloning the gene encoding emGFP amplified from pcDNA 6.2/C-EmGFP-DEST (Invitrogen) into pcDNA4/TO (Invitrogen) using KpnI and EcoRI restriction sites. pTetR was generated from pcDNA6/TR (Invitrogen). First, the XbaI site at 2509, bp in pcDNA6/TR was deleted by mutagenesis PCR using KAPA HiFi HotStart DNA (Kapa Biosystems) and a PstI site was added upstream of the blasticidin selection marker. The gene encoding eqFP650 was generated by oligo assembly PCR [55] and cloned into pcDNA6/TR using PstI and BlpI restriction sites, thus replacing the blasticidin cassette. pTetR − was constructed by deleting the TetR-encoding gene between the two BglII sites. ptTA was constructed by cloning tTA, amplified from pDM309 (ref. 56 ) (a generous gift of Dr Jeffrey Tabor), into pTetR using XbaI and EcoRI restriction sites. pTRE_tTA was generated by cloning the P TRE , consisting seven repeats of the 19 bp TO sequence and the CMV minimal promoter, which was amplified from pTreTight-Htt94Q-CFP (Addgene plasmid 23966), into ptTA using SpeI and HindIII restriction sites. TetR-CL1 and tTA-CL1 were generated by cloning the CL1 degron sequence [37] at the C terminal of TetR or tTA by three steps of reverse primer extension PCR. The cODC sequence [35] was constructed by oligo assembly PCR [55] and fused to the C terminal of TetR or tTA to generate TetR-ODC and tTA-ODC. TetR or tTA were replaced with TetR-CL1, TetR-ODC, tTA-CL1 or tTA-ODC in the plasmids pTetR, ptTA and pTRE_tTA using restriction sites EcoRI and BstXI to generate plasmids encoding the TetR and tTA variants. pPA28 was generated by cloning the PA28γ-encoding sequence, which was amplified from pOTB7 (Open Biosystems), into pcDNA3.1+ (Invitrogen) using KpnI and EcoRI restriction sites. Cell lines and transfections HeLa cells (the American Type Culture Collection) were cultured in EMEM, Lonza, supplemented with 10% fetal bovine serum (Sigma) and 1% penicillin–streptomycin–glutamine (Hyclone) and maintained at 37 °C and 5% CO 2 . Cells were harvested using trypsin (TrypLE, GIBCO Invitrogen). Cells were transfected using JetPrime (Polyplus transfection) according to the manufacturer’s protocol. Cells were transfected with the Deg-On system using a 1:6 ratio of pTO_GFP:pTetR and with the e Deg-On system using a 1:1:5 ratio of pTO_GFP:ptTA:pTRE_tTA. The culturing medium of transfected cells was replaced with fresh medium supplemented with MG-132 (Cayman Chemical) and/or tetracycline (Invitrogen) 24 h post transfection. The transfection conditions used in each experiment are reported in Supplementary Table 3 . The e Deg-On stable cell line was generated by first selecting a monoclonal stable population of HEK293 cells expressing TO_GFP. The plasmid pTO_GFP was linearized with FspI and transfected into HEK293 cells using JetPrime according to the manufacturer’s protocol. Stably transfected cells were selected using medium supplemented with zeocin (250 μg ml −1 ) for 3 weeks and subcultured into 96-well plates at a concentration of 0.5 cells per well to isolate monoclonal populations. A stable monoclonal cell line (HEK293/GFP) was selected for transfection with ptTA-CL1 and pTRE_tTA-CL1. The eqFP650 encoding cassette was replaced with the blasticidin-resistant gene in ptTA and with the puromycin-resistant gene in pTRE_tTA-CL1. ptTA and pTRE_tTA-CL1 were linearized using FspI and a 5:1 mixture (concentration ratio) was transfected into the HEK293/GFP cell line using JetPrime. Stably transfected cells were selected using blasticidin (5 μg ml −1 ) and puromycin (2 μg ml −1 ) for 3 weeks. A stable monoclonal cell line (HEK293/ e Deg-On) was isolated as described for HEK293/GFP cells. Western blot analyses Cells were lysed with Complete lysis-M buffer containing a protease inhibitor cocktail (Roche Applied Science) for 10 min. Lysed cells were centrifuged for 5 min at 14,000 g and 4 °C and supernatant was collected for western blot analyses. The protein concentrations were determined using the Bradford assay. Twenty micrograms of total proteins from each sample was separated by 10% SDS–PAGE. Western blots were conducted using mouse anti-TetR (MobiTech; 1:8,000), chicken anti-GFP (AnaSpec; 1:10,000), rabbit anti-glyceraldehyde 3-phosphate dehydrogenase (GAPDH; Santa Cruz Biotechnology; 1;8,000) and appropriate secondary antibodies (horseradish peroxidase-conjugated goat anti-mouse, goat anti-chicken and goat anti-rabbit (Santa Cruz Biotechnology; 1:12,000)). Blots were visualized using Luminata Forte Western HRP substrate (Millipore). Uncropped western blots images are reported in Supplementary Fig. 9 . Quantitative RT–PCR Total RNA was extracted using RNAGEM Tissue reagent (ZyGEM). Complementary DNA was synthesized from total RNA using qScript cDNA SuperMix (Quanta Biosciences) and quantified using a NanoDrop (Thermo Scientific). Quantitative PCR reactions were performed using PerfeCTa SYBR Green FastMix (Quanta Biosciences) in a CFX96 Real-Time PCR Detection System (Bio-Rad) with corresponding primers listed in Supplementary Table 4 . Samples were heated for 2 min at 95 °C and amplified using 45 cycles of 1 s at 95 °C, 30 s at 60 °C and 30 s at 72 °C. Analyses were conducted using CFX Manager software (Bio-Rad) and the threshold cycle (CT) was extracted from the PCR amplification plot [57] . The Δ C t value was used to describe the difference between the CT of a target gene and the CT of the housekeeping gene GAPDH and of the transfection control eqFP650 as follows: Δ C t =( C t (target gene)− C t (GAPDH))−( C t (eqFP650)− C t (GAPDH)). The relative mRNA expression levels of each sample were normalized to those of control cells consisting of untreated cells expressing TetR or tTA: relative mRNA expression level=2 [−(Δ C t_sample−Δ C t_control)] . Each data point was evaluated in triplicate and measured three times. Flow cytometry analyses Cells were analysed with a FACSCanto II flow cytometer (BD, San Jose, CA) to measure fluorescence intensity of GFP (488 nm laser, 530/30 nm emission filter) and eqFP650 (488 nm laser, 670/LP emission filter). At least 10,000 cells were recorded in each sample for analysis. For transient transfection experiments, we monitored changes in GFP signal within eqFP650-positive cells to monitor changes in GFP signal within transfected cells. The reported output signal was calculated by normalizing GFP to eqFP650 signal to eliminate differences arising from transfection efficiencies. Protein aggregation studies The APF was measured as previously described [58] , using the ProteoStat Aggregation detection kit (Enzo Life Sciences). The APF of cells expressing the eDeg-On system was calculated using the following formula: APF=100 × (MFI sample −MFI control )/MFI sample where MFI sample is the mean fluorescence intensity of the ProteoStat dye in HeLa cells transfected with the e Deg-On system (as described in the Results) and MFI control is the mean fluorescence intensity of control HeLa cells lacking both tTA and GFP and not treated with MG-132. Fluorescence intensity was measured by flow cytometry (488 nm laser, 585/40 nm emission filter). Statistical analyses All data are presented as the mean±s.d ( n ≥3 biological replica). Statistical significance was calculated using a two-tailed t -test in all experiments. Mathematical model GFP expression depends on GFP rate of synthesis ( R GFP_Syn ) and degradation ( γ GFP and on the rate of cell dilution ( μ ): The rate of GFP synthesis is described using the Hill function as previously described [59] modified to include GFP basal expression due to leakage [43] and to account for residual binding of tetracycline-bound TetR to TO: where β L is the GFP basal expression rate due to leakage, β GFPmax is the maximal synthesis rate, [TetR*] is the concentration of free TetR, K TetR is the dissociation constant of TetR binding to TO, [TetR −T c] is the concentration of TetR bound to tetracycline, K C is the dissociation constant of TetR−Tc binding to TO and n TetR is the degree of cooperativity of repression. TetR-tetracycline binding is also described using the Hill equation [31] : where [TetR] is the total cellular TetR concentration ([TetR]=[TetR*]+[TetR− T c]), [ T c] is the concentration of inducer (tetracycline), n Tc is the Hill coefficient of binding of tetracycline to TetR and K Tc is the concentration of tetracycline resulting in half-maximal binding. GFP expression (equation (1)) as a function of total TetR and tetracycline concentration was obtained using equations (2) and (3). It was previously reported that tetracycline diffuses through lipid bilayers very rapidly and without the aid of protein channels. As tetracycline diffusion equilibrium ( t 1/2 =35±15 min) [60] is reached much faster than steady-state GFP expression (30 h, Supplementary Fig. 1b ), the rate of tetracycline uptake was neglected. We assumed that the effect of UPS activity on the rate of degradation of GFP—a highly stable protein ( t 1/2 >24 h) [61] —is negligible compared with the effect of UPS activity on the rate of degradation of TetR. Thus, γ GFP was assumed to be constant. TetR expression (equation (4)) is defined in analogy to GFP expression (equation (1)) and depends on the rate of synthesis of TetR ( α ), which is constant, and on the rate of degradation of TetR ( γ TetR =ln2/ t 1/2 ). The half-life of TetR and, particularly, the half-life of TetR-Deg depend on UPS activity. Thus, TetR half-life was varied to simulate modulation of UPS activity. K Tc , K TetR , n Tc , n TetR , γ GFP and the dilution rate of HeLa cells ( μ ) were obtained from the literature ( Supplementary Table 1 ). The dissociation constant of TetR-tetracycline binding to TO ( K C ), TetR synthesis rate ( α ), TetR degradation rate ( γ TetR ) and GFP basal expression rate ( β L ) were estimated by fitting the experimental measurements of GFP fluorescence under the repression of wild-type TetR ( Fig. 1b ) to the steady-state model ( Supplementary Fig. 10 ) using nonlinear regression (MathWorks). The estimated value of K C was found to be five order of magnitude greater than the dissociation constant of TetR binding to TO ( K TetR ), in agreement with previously reported experimental studies [62] . To simulate self-activation of tTA expression, the equation describing tTA expression was modified to account for the rate of synthesis of tTA that is constitutively expressed ( α ′) and the rate of synthesis of tTA that is induced by tTA binding to its own promoter sequence ( ): The rate of tTA synthesis is described by the following Hill function: where is the maximum rate of synthesis of tTA self on self-activation, [tTA*] is the concentration of free tTA, is the dissociation constant of tTA binding to TO, [tTA− T c] is the concentration of tTA bound to tetracycline, K C is the dissociation constant of tTA-tetracycline binding to TO and is the Hill coefficient of binding of tTA to its own promoter DNA. The rate of tTA expression (equation (5)) as a function of total tTA and tetracycline concentration was obtained from equation (6). The rate of synthesis of GFP as a function of total tTA and tetracycline concentration was derived as described above for TetR and using the Hill function describing tTA binding. How to cite this article: Zhao, W. et al. Sensitive detection of proteasomal activation using the Deg-On mammalian synthetic gene circuit. Nat. Commun. 5:3612 doi: 10.1038/ncomms4612 (2014).